Comparative genome sequencing reveals genomic signature of extreme desiccation tolerance in the anhydrobiotic midge Anhydrobiosis represents an extreme example of tolerance adaptation to water loss, where an organism can survive in an ametabolic state until water returns. Here we report the first comparative analysis examining the genomic background of extreme desiccation tolerance, which is exclusively found in larvae of the only anhydrobiotic insect, Polypedilum vanderplanki . We compare the genomes of P. vanderplanki and a congeneric desiccation-sensitive midge P. nubifer . We determine that the genome of the anhydrobiotic species specifically contains clusters of multi-copy genes with products that act as molecular shields. In addition, the genome possesses several groups of genes with high similarity to known protective proteins. However, these genes are located in distinct paralogous clusters in the genome apart from the classical orthologues of the corresponding genes shared by both chironomids and other insects. The transcripts of these clustered paralogues contribute to a large majority of the mRNA pool in the desiccating larvae and most likely define successful anhydrobiosis. Comparison of expression patterns of orthologues between two chironomid species provides evidence for the existence of desiccation-specific gene expression systems in P. vanderplanki . Several organisms have evolved the ability to withstand extreme abiotic stresses, which are lethal for most other forms of life. Anhydrobiosis is a unique ametabolic state that enables a living organism to maintain viability even after losing more than 97% of its body water. Anhydrobiosis is generally associated with extraordinary cross-tolerance to a large variety of extreme conditions, such as temperatures ranging from −270 to +102 °C, vacuum and hydrostatic pressures up to 1.2 GPa and extremely high doses of radiation (up to 7,000 Gy) [1] , [2] . Anhydrobiotes also exhibit surprising longevity, and certain species have survived tens or even thousands of years in the dry form before recovery on rehydration [3] . Among metazoans, the ability to survive severe desiccation by entering an anhydrobiotic state is limited to several groups that include mostly microscopic organisms [1] . The largest and most complex anhydrobiotic animal is the larva of a non-biting midge, which is the sleeping chironomid Polypedilum vanderplanki [4] , [5] ( Fig. 1a ). Chironomid midges are known for their capacity to adapt to a wide variety of extreme environments and constitute a unique group among insects [6] . However, anhydrobiosis is a complex adaptive trait and de novo acquisition of such an extreme desiccation tolerance is most likely a unique evolutionary event. P. vanderplanki is the only anhydrobiotic species known to date among both chironomid midges and the entire insect lineage. In contrast to other anhydrobiotes (such as rotifers, tardigrades, nematodes or even plants) that are found in phyla showing widespread desiccation tolerance in a large array of species, P. vanderplanki is an isolated case among anhydrobiotes [1] . This finding suggests that the sleeping chironomid is a promising model for comparative genomics and should allow a precise dissection of the genetic background underlying the development of tolerance to complete desiccation. Over the last decade, investigations of the sleeping chironomid resulted in the identification of several groups of biomolecules, including late embryogenesis abundant (LEA) proteins, trehalose, antioxidants and heat–shock proteins contributing to desiccation tolerance [7] , [8] , [9] , [10] , [11] , [12] , [13] . In addition, in vitro and in vivo experiments have shown that these components are necessary but not sufficient to acquire complete desiccation tolerance. Therefore, whole-genome screening for anhydrobiosis-related features became an obligatory step in further understanding the molecular background of successful desiccation tolerance [14] , [15] . 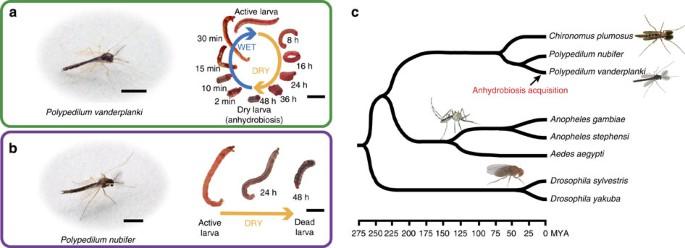Figure 1: Desiccation tolerance and phylogeny of two chironomid species. (a) Adult male of the sleeping chironomid,P. vanderplanki(left), and anhydrobiotic cycle of the larvae (right). During the dry season, larvae desiccate slowly to reach an ametabolic, quiescent state, termed anhydrobiosis. On rehydration, dried larvae rapidly recover normal activity. (b) Adult male of the congeneric chironomid,P. nubifer(left).P. nubiferlarvae can survive mild desiccation for 24 h like other chironomids, but they cannot enter anhydrobiosis and are killed by severe dehydration (right). Scale bar, 2 mm. (c) Phylogenetic tree inferred from the amino-acid sequence of cytochrome oxidase I (COI) showing the relationship betweenP. vanderplanki,P. nubiferand other Diptera. The scale shows the evolutionary distance between species in million years (MYA). Figure 1: Desiccation tolerance and phylogeny of two chironomid species. ( a ) Adult male of the sleeping chironomid, P. vanderplanki (left), and anhydrobiotic cycle of the larvae (right). During the dry season, larvae desiccate slowly to reach an ametabolic, quiescent state, termed anhydrobiosis. On rehydration, dried larvae rapidly recover normal activity. ( b ) Adult male of the congeneric chironomid, P. nubifer (left). P. nubifer larvae can survive mild desiccation for 24 h like other chironomids, but they cannot enter anhydrobiosis and are killed by severe dehydration (right). Scale bar, 2 mm. ( c ) Phylogenetic tree inferred from the amino-acid sequence of cytochrome oxidase I (COI) showing the relationship between P. vanderplanki , P. nubifer and other Diptera. The scale shows the evolutionary distance between species in million years (MYA). Full size image As mentioned above, the adaptation of P. vanderplanki is an isolated case of anhydrobiosis among all insects ( Fig. 1a ). A closely related species from the same genus, P. nubifer , is sensitive to desiccation ( Fig. 1b ). Thus, the combination of P. vanderplanki and P. nubifer represents a uniquely informative model of comparative genomics for deciphering the entire genetic background of anhydrobiosis. Our principal aim was to identify genome features specific to P. vanderplanki that are lacking in P. nubifer and other insects with sequenced genomes (including the fruit fly Drosophila and mosquitoes of the genera Anopheles and Aedes ; Fig. 1c ). This strategy allowed us to successfully identify several key genomic features accounting for extreme desiccation tolerance in P. vanderplanki . Among these features, the most obvious traits characterizing anhydrobiosis are the presence of specific genomic regions containing clusters of multi-copy protective genes involved in desiccation tolerance, the active utilization of protective proteins that most likely originate from horizontal gene transfer (HGT) and new desiccation-driven expression patterns for single genes that already exist in the P. vanderplanki genome. Assembly and characteristics of the chironomid genomes The ~600-fold coverage sequencing yielded a 104 Mbp for P. vanderplanki (scaffold N50=229 kbp) and 107 Mbp for P. nubifer (scaffold N50=26 kbp) genome assemblies ( Supplementary Note 1 ) approximating to the estimated genome sizes (96 and 95 Mb, respectively). A spread of metaphase giant chromosomes revealed a chromosome number of 2 n =8 for both species ( Supplementary Fig. 1 ). The P. vanderplanki genome is characterized by higher AT content and a low number of known transposable elements. The P. vanderplanki and P. nubifer genomes are predicted to contain 17,137 and 16,553 protein-coding loci, respectively ( Supplementary Note 1 ). The P. vanderplanki and P. nubifer genome contigs contain 97.18 and 95.56% of the complete core eukaryotic protein-coding sequences, which confirms the completeness of genome decoding ( Supplementary Note 1 ). The genome browser ‘MidgeBase’ containing both assembled contigs and mRNA-seq mapping data is accessible at http://bertone.nises-f.affrc.go.jp/midgebase ( Supplementary Fig. 2 ). The statistics of the assembled genomes are given in Table 1 . Table 1 The statistics of the assembled genomes of P. vanderplanki and P. nubifer . Full size table Gene expression in unstressed and desiccated larvae of both species The whole-genome transcription profile was different between two chironomid species in desiccation conditions. We estimated the InterProScan domains’ distribution in the proteins predicted to be expressed in the larvae of both species under unstressed conditions. As shown in Supplementary Table 1 and Supplementary Data 1 , the primary distribution of domains in P. vanderplanki and P. nubifer was similar. 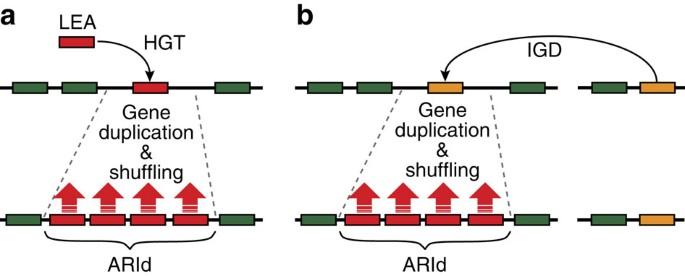Figure 2: Putative mechanism for the evolution of ARId in theP. vanderplankigenome. ARIds are genomic regions containing clusters of duplicated genes that are transcriptionally active during anhydrobiosis. (a) A gene of foreign origin (for example, LEA protein) is incorporated intoP. vanderplankigenome by HGT and undergoes extensive duplications and shuffling. (b) A pre-existingP. vanderplankigene originally not involved in anhydrobiosis and originating from another region ofP. vanderplankigenome was inserted to a new locus by intragenomic duplication (IGD) and undergoes extensive duplications and shuffling to acquire or improve a specific function for desiccation tolerance. All the genes in the ARIds from botha,bbecome highly upregulated during anhydrobiosis (red arrows). In contrast, a hypergeometric test (with confidence threshold P <1E−03) on the annotation of the distribution of the domains upregulated by desiccation for 24h (D24) in P. vanderplanki was exclusively enriched for thioredoxins (TRXs), protein-L-isoaspartate-(D-aspartate) O-methyltransferases (PIMTs), LEA proteins and globins ( Supplementary Table 2 ). Of the 100 P. vanderplanki genes showing the highest rate of upregulation during desiccation and abundance in the mRNA pool at different stages of dehydration, the majority are either represented by P. vanderplanki -specific loci (having no orthologue in P. nubifer or other insects) or was found within the top hits in the desiccation-specific domain-enrichment table ( Supplementary Table 2 ; Supplementary Data 2 ). Note that in P. vanderplanki , the upregulation of gene expression is observed throughout the desiccation process. However, transcriptional activity is most likely to be stopped completely when the dry anhydrobiotic state is reached (D48). Anhydrobiosis-Related gene Island (ARId) We noticed that in many cases, the genes encoding desiccation-specific mRNAs in P. vanderplanki are located in compact clusters in the genome. We defined P. vanderplanki -specific genomic regions where these gene sets are located as ‘anhydrobiosis-related gene island’ (ARId) to emphasize a possible contribution to desiccation tolerance. ARIds share the following common features ( Fig. 2 ): (a) they host a paralogous set of anhydrobiosis-related genes; (b) their localization in the genome is not necessarily related to that of the potential ancestor of the expanded set of genes; and (c) all genes located within ARIds are upregulated by desiccation [16] . Our current data suggest that the P. vanderplanki genome contains at least nine potential ARIds and each contains at least four paralogous highly desiccation-responsive genes (at least threefold increase in expression and RPKM (reads per kilo base of exon model per million mapped reads) value >10) in the cluster. In contrast, the P. nubifer genome contains no regions matching the ARId criteria. Figure 2: Putative mechanism for the evolution of ARId in the P. vanderplanki genome. ARIds are genomic regions containing clusters of duplicated genes that are transcriptionally active during anhydrobiosis. ( a ) A gene of foreign origin (for example, LEA protein) is incorporated into P. vanderplanki genome by HGT and undergoes extensive duplications and shuffling. ( b ) A pre-existing P. vanderplanki gene originally not involved in anhydrobiosis and originating from another region of P. vanderplanki genome was inserted to a new locus by intragenomic duplication (IGD) and undergoes extensive duplications and shuffling to acquire or improve a specific function for desiccation tolerance. All the genes in the ARIds from both a , b become highly upregulated during anhydrobiosis (red arrows). Full size image LEA protein genes located in ARIds LEA proteins possess chaperone-like or so-called molecular shield activity that protects proteins and membranes from desiccation stress [17] . They have been reported in both plants and invertebrates characterized by tolerance to water depletion [18] . Four genes encoding LEA proteins have been reported in P. vanderplanki [9] , [19] , but not in other insects (including insects with sequenced genomes). Analysis of the P. vanderplanki genome revealed 27 LEA protein genes ( Supplementary Data 3 ), but none in the P. nubifer genome ( Supplementary Data 3 ). These data suggest that the presence and activity of LEA proteins is correlated with anhydrobiotic capability. While plants have multigene families encoding LEA proteins (for example, 51 genes in Arabidopsis [20] ) of which the respective genes are distributed throughout the genome, only a few LEA proteins have been characterized in any particular invertebrate species [21] . At the same time, increasing numbers of transcriptome studies suggest that multiple LEA-like proteins are a feature of at least some anhydrobiotic animals [22] . P. vanderplanki genes encoding LEA proteins ( PvLea genes) are compactly arranged in two ARId clusters in the genome and there are some other genes interspersed [16] . None of the interspersed genes have orthologues in other insects or in P. nubifer . All predicted LEA-like genes in P. vanderplanki were expressed under non-desiccating conditions and most were strongly upregulated by desiccation ( Supplementary Data 4 ) [16] . In most cases, desiccated larvae contained the highest level of each PvLea mRNA and the mRNA expression returned to control levels in larvae rehydrated for 24 h ( Supplementary Data 4 ). To obtain insight into the possible origin of LEA protein genes in the P. vanderplanki genome, we conducted phylogenetic analyses using the BlastX protocol to identify homologies of PvLea genes with other insect genes. However, these analyses did not identify any homologues ( Supplementary Data 3 ). We expanded the search to other organisms and determined that the PvLea1 and PvLea5 genes (the largest length among Lea genes in P. vanderplanki ) had the highest similarity to LEA protein (Ce-LEA-1) from the nematode Caenorhabditis elegans and unknown protein (WP_020558683) from a soil bacteria Thiothrix flexiles , respectively ( Fig. 3 , Supplementary Data 3 ). We found the bacterial protein WP_020558683 significantly corresponded with PvLEA1 and PvLEA5 by comparing LEA proteins in P. vanderplanki using BlastP ( Supplementary Data 5 ). The Pfam search showed that both nematode- and bacterial-deduced proteins possessed several repetitions of an 11-mer amino-acid motif, so-called ‘LEA_4 motif (PF02987)’, which represent a feature of group 3 LEA proteins. On the basis of the studies on the properties of LEA proteins, it is known that their functional activity is defined by the repetitive 11-mer LEA motifs [23] . The motif search engine MEME SUITE [24] was then employed for further identification of repetitive amino-acid sequences in PvLEA1, PvLEA5 and WP_020558683. The search indicated that the distribution of the motifs in the PvLEA sequences resembled that of T. flexiles (a potential prokaryotic donor; Fig. 3 ). Both chironomid’s and the bacterial proteins had similar 11-mer motifs (motif 1 in Fig. 3 ), which were identical to the typical LEA motif [23] . These data imply that PvLea1 and PvLea5 were horizontally acquired from soil bacteria in the habitat of P. vanderplanki . The gene duplications and shuffling of these ancestral Lea genes within the P. vanderplanki genome may have generated the large PvLea cluster as an ARId ( Fig. 2a ). 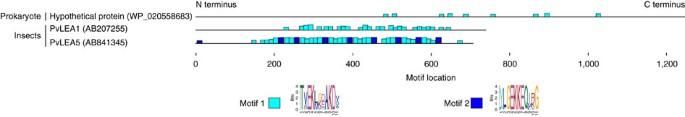Figure 3: Amino-acid motif distribution in PvLEA proteins and a bacterial hypothetical protein. The distribution was determined by MEME motif analysis (version 4.9.1). The closest non-eukaryotic genes resembling LEA proteins forP. vanderplankiand prokaryotes were identified by a cross-Blast search and used for analysis. The height of the motif block is proportional to –log(Pvalue), truncated at the height for a motif with aPvalue of 1e−10. MEME parameter settings were as follows: any number of repetitions for the distribution of motif occurrences; 11 for minimum and maximum motif width; and 2 for maximum number of motifs to find. Figure 3: Amino-acid motif distribution in PvLEA proteins and a bacterial hypothetical protein. The distribution was determined by MEME motif analysis (version 4.9.1). The closest non-eukaryotic genes resembling LEA proteins for P. vanderplanki and prokaryotes were identified by a cross-Blast search and used for analysis. The height of the motif block is proportional to –log( P value), truncated at the height for a motif with a P value of 1e−10. MEME parameter settings were as follows: any number of repetitions for the distribution of motif occurrences; 11 for minimum and maximum motif width; and 2 for maximum number of motifs to find. Full size image Antioxidants and ARId-specific TRXs Antioxidants play an important role in the adaptation to extreme dehydration in anhydrobiotes [25] . The expression of several key antioxidant genes is linked to anhydrobiosis in P. vanderplanki . Desiccated larvae accumulate corresponding mRNA and proteins so that during rehydration they can efficiently scavenge reactive oxygen species [13] . We identified 52 genes in P. vanderplanki and 29 genes in P. nubifer encoding core components of the insect enzymatic antioxidant systems [26] ( Supplementary Data 6 ). The number of such genes in P. nubifer is similar to that of other insects [26] . However, in P. vanderplanki , several groups of antioxidant genes have expanded ( Supplementary Data 6 ). In addition to the two cytoplasmic and single mitochondrial superoxide dismutases (SOD) that are well conserved among other insects including P. nubifer , the P. vanderplanki genome possesses two additional genes encoding a Zn-Cu-SOD ( Supplementary Data 6 ). On the basis of sequence similarity and genomic location, these genes are not paralogues of classical insect SOD. These SOD genes are highly expressed in response to desiccation and are most likely involved in anhydrobiosis ( Supplementary Data 7 ). Another remarkable finding is the appearance of additional exons in glutathione peroxidase genes that result in the formation of splice variants specifically upregulated in the cycle of anhydrobiosis (see Supplementary Note 2 and Supplementary Fig. 3 ). TRXs are small redox proteins present in all organisms [27] . These proteins are involved in redox signalling and act as antioxidants by facilitating the reduction of other proteins via cysteine thiol–disulfide exchange [28] . The number of TRXs in animal genomes ranges from one to five, and most isoforms are critical for normal organism function [29] . The two chironomid genomes both contain three TRXs that are well conserved in number and structure among insect genomes (insect TRX-1 to TRX-3 in Fig. 4a ). However, the P. vanderplanki genome contains 21 additional genes encoding TRXs arranged in two ARIds unlinked to the classical TRX set of genes ( P. vanderplanki -specific TRX in Fig. 4a ; Supplementary Data 6 and 8 ). These newly identified TRXs share key features of cytosolic TRX, including small size and a single TRX domain. In addition, all of the genes are strongly upregulated by desiccation. In contrast, the classical TRX genes in P. vanderplanki ( PvTrx1–3 ) respond only moderately to water loss ( Supplementary Data 7 ). 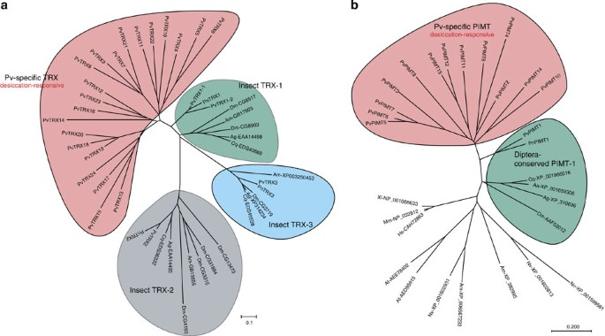Figure 4: Evolutionary relationships of the classical and novel desiccation-responsive TRX and PIMT proteins. (a) Phylogenetic tree of TRX proteins showing the clusters of classical insect TRX-1 (green), TRX-2 (grey), TRX-3 (blue) and the cluster of desiccation-responsive TRX, specific toP. vanderplanki(pink). (b) Phylogenetic tree of PIMT proteins showing the cluster of the classical PIMT-1 conserved among Diptera (green) and the cluster of desiccation-responsive PIMT proteins, which are specific toP. vanderplanki(pink). The evolutionary history was inferred using the neighbor-joining method and the evolutionary distances were computed using the maximum likelihood estimation (units: amino-acid substitutions per site). Pv,P. vanderplanki; Pn,P. nubifer; Aa,Aedes aegypti; Ag,Anopheles gambiae; Am,Apis mellifera; Cq,Culex quinquefasciatus; At,Arabidopsis thaliana; Dm,Drosophila melanogaster; Hs,Homo sapiens; Mm,Mus musculus; Nv,Nasonia vitripennis; XI,Xenopus laevis. Figure 4: Evolutionary relationships of the classical and novel desiccation-responsive TRX and PIMT proteins. ( a ) Phylogenetic tree of TRX proteins showing the clusters of classical insect TRX-1 (green), TRX-2 (grey), TRX-3 (blue) and the cluster of desiccation-responsive TRX, specific to P. vanderplanki (pink). ( b ) Phylogenetic tree of PIMT proteins showing the cluster of the classical PIMT-1 conserved among Diptera (green) and the cluster of desiccation-responsive PIMT proteins, which are specific to P. vanderplanki (pink). The evolutionary history was inferred using the neighbor-joining method and the evolutionary distances were computed using the maximum likelihood estimation (units: amino-acid substitutions per site). Pv, P. vanderplanki ; Pn, P. nubifer ; Aa, Aedes aegypti ; Ag, Anopheles gambiae ; Am, Apis mellifera ; Cq, Culex quinquefasciatus ; At, Arabidopsis thaliana ; Dm, Drosophila melanogaster ; Hs, Homo sapiens ; Mm, Mus musculus ; Nv, Nasonia vitripennis ; XI, Xenopus laevis . Full size image Unexpected diversity of protein-repair methyltransferases in ARId PIMT is an enzyme that recognizes and catalyses the repair of damaged L -isoaspartyl and D -aspartatyl groups in proteins [30] . PIMT partially restores aspartic residues in proteins that have been non-enzymatically damaged due to age and extends the life of its substrates. This highly conserved enzyme is present in nearly all eukaryotes, Archaea and gram-negative eubacteria mostly as a single isoform (or as a few isoforms in certain plants and some bacteria) [31] . Insects have a single copy of the PIMT-coding gene like plants, nematodes and mammals. PIMT activity in animals was found to be tightly linked to stress resistance and lifespan [30] , [31] . The structure and number of PIMT-coding genes in the two chironomid species varied dramatically. Both species have the orthologues of PIMT shared by dipteran insects (PIMT-1 in Fig. 4b ; Supplementary Data 9 ). P. nubifer has only one PIMT gene ( PnPimt1 ). However, the P. vanderplanki genome contains 13 additional genes paralogous to Pimt1 ( PvPimt2–14 in Fig. 4b ). These genes presumably code for functional PIMT proteins. The genes are arranged in a single cluster [16] . Remarkably, the PvPimt1 location in P. vanderplanki is not within the single ARId constituting other Pimt -like genes. The expression of PIMT1-coding gene in both chironomids ( PvPimt1 and PnPimt1 ) did not change in response to desiccation, but the clustered PvPimt2–14 genes showed upregulation on entering anhydrobiosis ( Supplementary Data 9 ). The abundance of PvPimt2–14 mRNAs was maximal in anhydrobiotic larvae and resembled plant seeds where the accumulation of PIMT provides additional protection for proteins during long periods of dry storage by exerting their repair function on rehydration [32] . The predicted proteins corresponding to PvPimt2–14 contain the conserved PIMT functional domain. In addition, the length and structure of the amino- and carboxy-terminal regions of the predicted proteins show marked variation. These findings suggest different substrate preferences or other specific properties of the various PvPIMTs. This multi-member family in P. vanderplanki is the first observation of large-scale expansion of Pimt genes in general and has not been reported in a single insect species. Haemoglobins and anhydrobiosis Chironomids are the only group of insects with haemolymph haemoglobins (Hbs) that act as the main respiratory proteins. Thus, chironomid Hbs have a respiratory function analogous to vertebrate Hb. Hbs enhance the O 2 capacity of the haemolymph and enable O 2 transport in the larvae. In addition, Hbs are also assumed to be involved in oxygen storage during periods of hypoxia in poorly aerated water [33] . The genomes of the two Polypedilum species contain multiple Hb homologues which form several gene clusters. We have identified 33 and 25 Hb genes in the P. vanderplanki and P. nubifer genome, respectively. This study is the first complete genome-based survey of chironomid globins. The structure (represented by both intron-less and intron-bearing orthologues) and multiple nature of the PvHbs gene family is similar to that of P. nubifer and other midge species [33] . However, while the activity of Hb is believed to be mostly larval stage specific, we found that three PvHb genes ( PvHb11, 12 and 21 ) are exclusively expressed in eggs. This expression is not maternally acquired from adult haemolymph (see MidgeBase browser) as previously suggested [33] . Another remarkable difference between the two Polypedilum species is that the increased number of Hb genes in P. vanderplanki results from the insertion of a new cluster of paralogous intron-less Hb genes located in an ARId consisting of six members (see ARId sub-genome browser [16] ). This gene set ( PvHb11, 12, 17, 23, 24, 25, 32 and 33 in Supplementary Data 10 ) is strongly upregulated on desiccation. In contrast, all PnHb genes and their orthologous counterparts in P. vanderplanki are downregulated in the desiccating larvae ( Supplementary Data 10 ) [33] . Four of the 6 anhydrobiotic chironomid-specific Hb genes ( PvHb17, 23, 32 and 33 ) also showed high mRNA levels under non-stressed conditions and are 4 of the 10 most highly expressed Hb genes in the wet larvae ( Supplementary Data 10 ). Our data on developmental stage-specific and anhydrobiosis process-specific patterns of Hb gene expression suggest that the multiple members of this gene family in the chironomids are most likely involved in specialization of the function rather than a general increase in Hb protein dosage, as proposed by some authors [33] . One possibility is that the P. vanderplanki -specific Hbs may have specific properties allowing them to provide effective delivery of oxygen under conditions of increased molecular crowding in the larvae due to desiccation. Alternatively, the Hbs may protect larvae against free radicals generated during severe dehydration. Other examples of the process generating ARIds in P. vanderplanki genome ( Fig. 2b ) are gene clusters coding small heat–shock proteins and several unknown genes [16] . Aquaporins and dehydration process en route to anhydrobiosis Water channels or aquaporins (AQPs) primarily control permeation of water across the phospholipid bilayer of the cell membrane [34] . Thus, AQPs most likely play pivotal roles in the dehydration process en route to anhydrobiosis. We have identified five AQP-coding genes in each species of the chironomid ( Aqp1–5 ; Supplementary Table 3 ), which is a similar number to other dipteran insects [35] , [36] . Aqp1 encodes the water-specific AQP and showed differences in the mRNA-level response to desiccation between the two species. In the anhydrobiotic species, the corresponding gene was strongly responsive to desiccation and its expression increased by more than threefold. The mRNA for Apq1 represented more than 80% of all AQP mRNAs in the larvae subjected to slow desiccation. In contrast, expression of Aqp1 in P. nubifer under desiccation did not increase ( Supplementary Table 3 ). Aqp1 was previously assumed to play a key role in trafficking water out of the body of the anhydrobiotic P. vanderplanki larvae [37] . The current comparative analysis of P. vanderplanki and P. nubifer Aqp1 orthologues revealed evolution of specific mRNA regulation in response to desiccation. In P. vanderplanki , the total abundance of Aqp1 mRNA in the larvae was higher under normal conditions and further drastically increased under slow desiccation ( Supplementary Table 3 ). Anhydrobiosis-related trehalose metabolism pathway Trehalose is a disaccharide of glucose that stabilizes intact cells in the dry state and replaces water [1] , [7] , [38] . P. vanderplanki larvae synthesize large amounts of trehalose (up to 20% dry mass) during dehydration en route to anhydrobiosis [1] , [8] . In dehydrated larvae, trehalose stabilizes the structure of biomolecules [38] . Recently, we isolated genes coding for trehalose-6-phosphate synthase (TPS) and trehalose-6-phosphate phosphatase (TPP). These genes govern trehalose synthesis and trehalase (TREH) hydrolyses trehalose into its component glucose units [11] . Trehalose is abundantly synthesized from glycogen in the fat body in response to water loss. The elevated sugar concentration is achieved by increased TPS and TPP activities and suppression of TREH activity [11] . In addition, in P. vanderplanki , TRET1 facilitates the transport of trehalose across cellular membranes of the fat body cell [10] . TRET1 retains a high capacity for transport activity even when trehalose is highly concentrated in the dehydrating larval body during the final stage of entry into anhydrobiosis [10] . In both chironomids, the genes encoding members of the trehalose metabolism pathway (TMP) including TRET1, TPP, TPS and TREH are represented by single-copy genes ( Supplementary Table 4 ) that are similar to those of other insects both in sequence and gene structure. However, the TMP genes in the two chironomid species responded very differently to desiccation. The expressions of both TPS and TREH were drastically elevated in P. vanderplanki but remained unchanged in P. nubifer . In contrast, the genes encoding TRET1 and TPP in both species showed a similar pattern of expression and were slightly increased in response to desiccation ( Supplementary Table 4 ). These data suggest that in P. vanderplanki , the accumulation of trehalose during the onset of anhydrobiosis is mediated not by a special set of genes (the number and structure of TMP genes in P. vanderplanki is similar to that of other insects), but rather by the evolution of gene expression control mechanisms responsive to desiccation. Another important question is how a simultaneous increase in TREH mRNA and protein [11] in the larvae could be associated with a general decrease in the activity of this trehalose-hydrolysing enzyme. Post anhydrobiosis, the rapid decrease in trehalose concentration in the larvae is mediated by TREH activity. Our previous data suggest that the enzyme is stored in the larvae in advance of its requirement during rehydration [11] . As mentioned above, TRET1 has a pivotal role for transport of trehalose synthesized in the fat body in the desiccating larvae [10] . Other desiccation-inducible transporters might be involved in trehalose uptake in the peripheral tissues on dehydration (see Supplementary Note 3 ; Supplementary Table 5 ). Elucidating the origins of ARIds and the amplification of genes in these regions are critical for understanding the genomics of anhydrobiosis. Desiccation causes extensive DNA damage and anhydrobiotic larvae require several days to repair the damage following rehydration [13] . This DNA damage likely increases the frequency of genome rearrangements. Furthermore, cycles of anhydrobiosis might promote HGT as suggested for rotifers [39] . A preliminary analysis identified at least 12 expressed genes in the P. vanderplanki genome with strong evidence for HGT and these genes are mostly from prokaryotes ( Supplementary Table 6 ). The hypothetical scenario of HGT would be an integration of foreign DNA to the genome of the chironomid from consumed bacteria because it is the primary food source of the larvae. In addition, potential disruptions of cell membranes and severe DNA fragmentation associated with every cycle of anhydrobiosis [13] are likely to facilitate this process. The AQP and TMP genes are not located in ARId regions, but show desiccation-responsive expression patterns that are similar to what is observed with the genes from ARId clusters. Examining the P. vanderplanki genome and comparing ARIds and AQP or TMP gene-coding regions are promising models for uncovering the structure of yet unknown desiccation-inducible cis -elements and/or trans -regulation modules such as transcription factors and noncoding RNAs. In summary, anhydrobiosis-associated genes (including chaperone-like proteins, antioxidants, aging-related proteins and unique globins) in P. vanderplanki have undergone massive expansion within the gene clusters or ARIds [16] . For example, phylogenetic analysis of PvLea genes shows that the majority have no significant similarity (BlastP bit score <100) to LEA protein genes in other organisms and most likely resulted from extensive gene duplication after a founding HGT event ( Fig. 2 ; Supplementary Data 5 ). Finally, an important event for the evolution of anhydrobiosis in P. vanderplanki is the acquisition of new regulatory pathways that are strongly responsive to desiccation. These regulatory pathways control the expression of the gene clusters located in ARId regions and also control isolated genes co-opted for anhydrobiosis (TMP or AQP genes). All these evolutional changes are likely to be further mediated by P. vanderplanki ecology and DNA-damaging effects of desiccation. The nature of P. vanderplanki habitats (large isolated rocks), the poor flying ability and strong selection pressure due to the long dry season in semi-arid areas of Africa facilitated microevolutionary patterns in this species. Our recent in vitro data show the direct contribution of the members in the expanded gene clusters (such as LEA proteins and antioxidants) to neutralize the effects of desiccation. Another possibility is a non-adaptive gene drift-based origin of the observed changes in P. vanderplanki genome. Future comparative investigations on isolated P. vanderplanki populations will certainly help to verify these hypotheses for the de novo acquisition and the evolution of anhydrobiosis in this unique insect. Insects Highly inbred lines of these sibling species that differ in their ability to resist complete desiccation were used for genomic DNA extraction. P. vanderplanki and P. nubifer larvae were reared on a 1% agar diet containing 2% commercial milk under controlled photoperiod (13 h light: 11 h dark) and temperature (27–28 °C) conditions. Number of chromosomes of P. vanderplanki and P. nubifer We observed polytene chromosomes in the salivary glands of fully hydrated larvae of P. vanderplanki and P. nubifer . Fourth instar larvae were fixed in a 3:1 mixture of 96% ethanol and glacial acetic acid and stored at −80 °C until use. Salivary glands were dissected out and stained in 1.0% orcein in 45% acetic acid. They were then washed lightly in 45% acetic acid and squashed in 50% lactic acid. Estimation of the chironomids’ genome sizes by flow cytometry The genome sizes of the two species were determined by flow cytometry (Cornette et al ., in prep). Briefly, heads of adult chironomids were homogenized into a solution of 0.5% Triton X-100 in 1 ml phosphate buffered saline buffer, before staining the nuclei with 5 μg ml −1 of propidium iodide and filtering on a 30-μm mesh filter (Partec, Münster, Germany). The DNA content of stained nuclei was measured by a Coulter Epics Elite flow cytometry system (Beckman Coulter, Indianapolis, IN). The 2C DNA content of the sample was compared with the standard 0.36 pg DNA of D. melanogaster diploid nuclei. Genomic DNA sampling Genomic DNA from over 500 final instar larvae (of ~1 mg wet body weight) for construction of mate-pair libraries and other experiments was isolated with conventional cetrimonium bromide (CTAB) method [40] and NucleoSpin tissue (Macheley-Nagel, Düren, Germany), respectively. Genome sequencing Genome sequences were obtained using paired-end and mate-pair protocols on Illumina HiSeq 2000, GAIIx and SOLiD 4 instruments. Genomic DNA was fragmented, libraries prepared and sequencing conducted according to the manufacturer’s protocols. Mate-paired libraries for the SOLiD 4 system (Life Technologies, Carlsbad, CA) with inserts of ~2.5 kb were constructed from 5 μg of genomic DNA, and deposited on two quarters of a flow cell for each sample. Fifty base reads were obtained from each of the F3 and R3 tags, with 22 Gbp for both P. vanderplanki and P. nubifer libraries. To construct the libraries for whole-genome sequencing, DNA was processed using a TruSeq DNA Sample Preparation kit v.2 (Illumina, San Diego, CA) according to the manufacturer’s instructions. Library lengths, as assessed using an Agilent 2100 Bioanalyzer (Agilent Technologies, Santa Clara, CA), were 541 for P. nubifer and 397 for P. vanderplanki . Libraries were quantified using fluorometry with Qubit 2.0 (Life Technologies) and real-time PCR, and diluted to final concentration of 9 pM. Diluted libraries were clustered using a cBot instrument (Illumina) with a TruSeq PE Cluster Kit v3 (Illumina) and sequenced using a HiSeq 2000 sequencer (Illumina) with TruSeq SBS Kit v3-HS (Illumina), read length 101 from each end. Poly A-mRNA libraries were constructed using TruSeq RNA Sample Preparation kit v.2 (Illumina) and quantified and sequenced in the same way as genomic DNA libraries. For the P. vanderplanki genome, sequencing with a single-molecule real-time sequencer was also performed. Approximately 6- and 10-kb insert libraries were constructed and sequenced with C2 chemistry using PacBio RS (Pacific Bioscience, Menlo Park, CA) for 34 cells (version 2). Using two types of libraries, the GAIIx platform generated a total of 36.8 Gbp of P. vanderplanki sequence data ( Supplementary Table 7 ). Furthermore, the HiSeq 2000 platform produced 6.9 Gbp of sequence data, the SOLiD 4 system generated 20.9 Gbp data and the PacBio RS yielded 1,479,033 reads with 1.7–2.7 kb mean maximum subread length, total 2.9 Gbp of independent fragment reads. On the basis of the genome size estimation of 100 Mbp (see above), the total of 67.5 Gbp of sequence data obtained corresponds to ~562-fold coverage of the P. vanderplanki genome ( Supplementary Table 7 ). In the case of P. nubifer , the HiSeq 200 platform generated 7.0 Gbp sequence data, providing ~58-fold coverage of that chironomid genome ( Supplementary Table 8 ). Genome sequence assembly The shotgun, paired-end and mate-pair reads were assembled de novo by the Platanus Assembler [41] ( http://platanus.bio.titech.ac.jp ) and the remaining gaps were filled with PacBio RS reads using the PBJelly pipeline [42] . Fosmid-end sequences The fosmid library of P. vanderplanki genome was prepared by Takara Bio (Shiga, Japan). Randomly selected fosmid clones were end sequenced by the Sanger method using an ABI 3130xl sequencer (Life Technologies). Evaluation of assembly with core eukaryotic genes Gene coverage of the P. vanderplanki and P. nubifer genome assemblies was evaluated with 248 core eukaryotic genes using CEGMA 2.4 (Core Eukaryotic Genes Mapping Approach) [43] . Repetitive and transposon-like regions in the genomes We ran RepeatModeler [44] with default parameters to identify de novo repeat elements and classify them automatically. The programme internally incorporates three de novo repeat finders, that is, RECON [45] , RepeatScout [46] and TRF (Tandem Repeat Finder) [47] and generates libraries of repeat sequences. Transcriptome sequencing and mapping Transcriptome analysis is essential to understand gene expression profiles in specific organisms. For more effective prediction of the gene models and genetic network associated with desiccation resistance, we performed complex mRNA expression analysis of the two chironomids, combining known expressed sequence tag (EST) databases [48] and newly prepared data with the aid of next-generation sequencing technologies. We obtained 454 ESTs from the P. vanderplanki complementary DNA (cDNA) library using the 454 GS FLX Titanium platform (454 Life Science, Branford, CT). The cDNA library for 454 ESTs was prepared according to Meyer et al . [49] and sequenced according to manufacturer’s instructions. A total of 885,642 reads, with an average length of 355 bp, resulted in over 314 Mbp of data. Before downstream analysis, adaptor and vector sequences in the raw tags were trimmed with SeqClean [50] software and UniVec database [51] . This pre-process resulted in 852,333 high-quality reads with a minimum length of 100 bp. High-throughput mRNA sequencing (RNA-seq) offers the ability to discover new genes and transcripts and measure transcript expression in a single assay. To develop comprehensive insight into differential gene expression during dehydration and rehydration and to improve coverage of transcriptome data, we performed deep RNA sequencing from various RNA samples. Total RNA from four hydrated, dehydrating and rehydrated ( P. vanderplanki only) larvae (each of 50 individuals) was extracted using Trizol (Life Technologies) and the RNeasy Mini Kit (Qiagen, Hilden, Germany), according to the manufacturer’s recommendations. TruSeq RNA Sample Preparation kit v.2 (Illumina) was used for preparation of RNA-seq libraries. For P. vanderplanki , RNA was collected from whole larvae at 0, 24 and 48 h of dehydration (each of 50 individuals). RNA was also sampled from whole larvae at 3 and 24 h after rehydration. For P. nubifer , RNA was sampled from whole larvae only at 0 and 24 h of dehydration (each 50 individuals). These samples were subjected to deep sequencing on the Illumina GA II platform. In the same manner, RNA from four life stages (eggs, larvae, pupae and adults) for P. vanderplanki and one stage (larvae) for P. nubifer was extracted and sequenced on the Illumina HiSeq 2000 platform. RNA-seq reads’ source data are summarized in Supplementary Table 9 . Gene prediction Gene model predictions were generated using AUGUSTUS software (version 2.6.1) [52] , [53] . Because of the unavailability of species parameters for P. vanderplanki and P. nubifer , we first trained AUGUSTUS to create the parameter sets for both species. We adopted iterated training using predicted genes generated with the existing parameter set for Anopheles gambiae . After iterated training, parameters were adjusted with the built-in Perl script, optimize_augustus.pl, to optimize prediction accuracy. We also constructed extrinsic evidence about genes from available transcriptome data, including Sanger ESTs, 454 ESTs and RNA-seq reads. Sanger ESTs were mapped onto genomic sequences using GMAP [54] . ESTs from the 454 FLX platform were assembled into contigs using MIRA3 (ref. 55 ) before the mapping process and were aligned to the genome with BLAT [56] . RNA-seq reads were assembled into transcripts using TopHat2 (ref. 57 ) and Cufflinks [58] . Protein genome alignment data between A. gambiae and Aedes aegypti protein and genomic sequences, generated with Exonerate [59] , were also incorporated. The complete data set was merged into a ‘hint file’ and used for gene prediction. The resultant numbers of genes for P. vanderplanki and P. nubifer were 17,824 and 17,224, respectively. All RNA-seq reads ( Supplementary Table 9 ) were mapped onto gene models using Bowtie2 (ref. 60 ) with default parameters to estimate expression level (RPKM). We filtered out all genes with either an RPKM value of 0 or a raw tag count below 2 in all samples. This process discarded 207 and 394 genes of P. vanderplanki and P. nubifer , respectively. Transposable element-derived proteins were also filtered out based on automated annotation results, including InterProScan and BlastP (1e−05, no filter). The final P. vanderplanki gene model set contained 17,137 genes and the final gene model set for P. nubifer consisted of 16,553 genes ( Supplementary Table 10 ). Identification of chironomid genes Predicted genes were annotated using a set of publicly available tools. We performed BlastP (version 2.2.25) [61] searches of gene models against NCBI-nr with an expectation value of 1.0e−05. As a result, for P. vanderplanki and P. nubifer , 2,558 out of 14,579 (17.5%) and 3,201 out of 13,352 (24.0%) genes did not have a significant hit, respectively. Protein domain annotation of gene models was done by combination of HMMER3 and domain models’ Pfam A [62] , [63] . To obtain more comprehensive information on protein function, all deduced proteins were subjected to InterProScan (version 4.8) analysis. The result of annotation for all P. vanderplanki and P. nubifer genes, together with the expression data (RPKM), was prepared as a single MS-Excel file ( Supplementary Data 11 ). The frequency of Gene Ontology terms and InterPro IDs [64] for P. vanderplanki and P. nubifer were also summarized ( Supplementary Data 1 ). Estimation of expression of the predicted genes The mRNA expression levels for the entire transcript set ( Supplementary Table 9 ) were estimated using the RPKM values. For confident comparison of the transcriptional response to desiccation in the two chironomids, only two sets of data (wet larvae versus larvae desiccated for 24 h, termed D0 and D24) were used. An increase in expression of more than threefold and an RPKM value >10 for the higher value were used as the criteria for placement of a gene in the ‘desiccation-responsive’ group. The expression data were represented by tracks in the genome browser. Genome browser A genome browser for the assembled genome sequences has been established using the Generic Genome Browser (GBrowse) 2.17 (ref. 65 ) ( Supplementary Fig. 2 ), incorporating both the genome structure of the two chironomid species and genome-wide mRNA expression data in response to desiccation ( P. nubifer ) and for the complete cycle of anhydrobiosis ( P. vanderplanki ). The URL for the browser is: Midgebase http://bertone.nises-f.affrc.go.jp/midgebase ; GBrowse for P. vanderplanki http://bertone.nises-f.affrc.go.jp/cgi-bin/gb2/gbrowse/pv091 ; GBrowse for P. nubifer http://bertone.nises-f.affrc.go.jp/cgi-bin/gb2/gbrowse/pn090 ; and GBrowse for ARIds http://bertone.nises-f.affrc.go.jp/cgi-bin/gb2/gbrowse/arid/ . Alignment of the sequences and building the phylogenetic trees A phylogenetic tree of P. vanderplanki in dipteran species inferred from the amino-acid sequence of cytochrome oxidase I (COI) was adapted from several previous analyses [66] , [67] , [68] , [69] . The deduced protein sequences were used to reconstruct phylogeny of TRX and PIMT in P. vanderplanki and P. nubifer . The alignment was done using MUSCLE [70] in CLC Main Workbench 6 (CLC bio, Aarhus, Denmark) and the trees were built using neighbour joining with 1,000 bootstraps. The reference orthological genes from other insects were derived from the public database. Pipeline for identification of horizontally transferred genes We used a custom phylogenomic pipeline to build gene trees for all predicted coding regions in P. vanderplanki and P. nubifer ; scripts are available from the authors on request. Predicted amino-acid sequences were first queried using BlastP against a local database consisting of NCBI’s Reference Sequence and predicted protein sequences from recently sequenced microbial eukaryotes (JGI genome portal and Ghent University’s online genome annotation server BOGAS). For each Blast result, a hit was considered significant if the E -value was ≤1e−3, the bit score was ≥60 and fraction conserved was ≥0.3. If a hit met these sequence similarity thresholds, the associated sequence was extracted from the database using a custom Perl script. To reduce the number of paralogues in the analysis, only the top four hits per species were extracted. Extracted sequences were reordered based on global similarity to the query sequence with MAFFT using the minimum linkage clustering method and rough distance measurement (number of shared 6-mers) [71] . After reordering, the files were reduced to include only the top 200 sequences, and files with fewer than 4 sequences were eliminated. Alignments were performed with MAFFT using the automated strategy selection. Poorly aligned positions and sequences were removed from the alignment using REAP [72] , and trimmed alignments were further refined by a second MAFFT alignment using the same parameters as above. Phylogenetic trees were inferred using FastTree, assuming a JTT+CAT amino-acid model of substitution and 1,000 bootstrap replicates [73] . For each tree, the phylogenetic sister group to Polypedilum was determined using SICLE [74] ( http://eebweb.arizona.edu/sicle/ ). Finally, the candidate genes were analysed manually to filter out potential false-positive cases. The results of final screening are summarized in Supplementary Table 6 . How to cite this article: Gusev, O. et al . Comparative genome sequencing reveals genomic signature of extreme desiccation tolerance in the anhydrobiotic midge. Nat. Commun. 5:4784 doi: 10.1038/ncomms5784 (2014). Accession codes: Sequence data for P. vanderplanki and P. nubifer have been deposited in GenBank/EMBL/DDBJ nucleotide core database under the accession codes PRJDB1558 and PRJDB2914 , respectively.